Copy number variation of the restorerRf4underlies human selection of three-line hybrid rice breeding Cytoplasmic male sterility (CMS) lines are important for breeding hybrid crops, and utilization of CMS lines requires strong fertility restorer ( Rf ) genes. Rf4 , a major Rf for Wild-Abortive CMS (CMS-WA), has been cloned in rice. However, the Rf4 evolution and formation of CMS-WA/ Rf system remain elusive. Here, we show that the Rf4 locus emerges earlier than the CMS-WA gene WA352 in wild rice, and 69 haplotypes of the Rf4 locus are generated in the Oryza genus through the copy number and sequence variations. Eight of these haplotypes of the Rf4 locus are enriched in modern rice cultivars during natural and human selections, whereas non-functional rf4i is preferentially selected for breeding current CMS-WA lines. We further verify that varieties carrying two-copy Rf4 haplotype have stronger fertility restoration ability and are widely used in three-line hybrid rice breeding. Our findings increase our understanding of CMS/ Rf systems and will likely benefit crop breeding. Cytoplasmic male sterility (CMS), a maternally inherited trait caused by mitochondrial gene rearrangement and the interaction between mitochondrial genes and nuclear genes, occurs widely in plants [1] , [2] , [3] . The discovery of CMS and fertility restorer ( Rf ) genes in rice ( Oryza sativa ) enables the production of hybrid rice using a three-line system, a successful model for utilizing heterosis to improve rice yield [3] . Three major types of CMS systems have been used in three-line hybrid rice breeding: Wild Abortive type (CMS-WA) [4] , HongLian type (CMS-HL) [5] , and Boro II type (CMS-BT) [6] . Three-line hybrid rice production in China primarily uses CMS-WA rather than CMS-HL and CMS-BT (1983–2018) [7] , [8] ( http://www.ricedata.cn/ ). Because three-line hybrid rice production requires restoration of fertility in CMS, understanding the evolution and selection of related Rf genes provides important information for facilitating and potentially improving hybrid rice breeding. The Oryza genus, including 25 wild species and 2 cultivated species (Asian cultivated rice O. sativa and African cultivated rice O. glaberrima ), has undergone significant diversification over the course of evolution, with many of Oryza species diverging within the past 15 million years [9] , [10] . Asian cultivated rice is divided into two subspecies: O. sativa indica and O. sativa japonica [11] , [12] , [13] . The CMS-WA lines were developed by introgressing CMS cytoplasm from common wild rice ( O . rufipogon ) into some indica rice cultivars [4] . We previously cloned the CMS-WA gene WA352 , which encodes a cytotoxic mitochondrial protein that causes premature programmed cell death in anther tapetum cells, ultimately leading to pollen abortion [14] . According to our evolutionary analysis, the mitochondrial gene WA352 (renamed WA352c [1] ) is a newly formed CMS gene derived from non-functional CMS-like protogenes ( orf356 and orf367 ), through multiple rearrangements of mitochondrial genome sequences accompanied by sub-stoichiometric shifting, sequence variation, and natural selection in O . rufipogon [1] . We also cloned one of the major CMS-WA restorer genes, Rf4 [15] ; the other CMS-WA restorer gene, Rf3 , remains to be cloned [16] . Rf4 encodes a pentatricopeptide repeat (PPR) protein of 782 amino acids, which restores CMS-WA fertility by mediating degradation of the WA352 mRNA [15] . Although we and other groups previously identified five variants of Rf4 ( Rf4 M [haplotype H1], Rf4 I [H2], H3 [ rf4aus , see below], rf4i [H4], and rf4j [H5]) [15] , [17] , [18] , the evolutionary trajectory of Rf4 in the Oryza genus is unclear, and how the CMS-WA gene WA352c co-evolved with the functional Rf4 gene during natural and human selections remains unknown. Most Rf genes in plants encode P-type PPR proteins function as sequence-specific RNA binding proteins to destroy the functions of newly emerging mitochondrial CMS genes, a process that might be driven by selection [19] , [20] , [21] . PPR genes often occur in clusters and PPR genes within these clusters show high sequence similarity; these clusters may form through tandem duplication, thus contributing to expansion of the PPR gene family [22] . For example, a PPR gene cluster on rice chromosome 10 consists of at least ten PPR genes within an about 400-kb region (according to the reference genome of a restorer line MH63 (Minghui63, fertility restorer line carrying functional Rf4 , http://rice.hzau.edu.cn/rice_rs3/ ) [23] , including Rf4 for CMS-WA [15] , Rf1a and Rf1b for CMS-BT [24] , Rf5 for CMS-HL [25] , and Rf19 for CMS-FA [26] . The PPR genes in the Rf4 locus have evolved rapidly through sequence duplication and allelic variation, generating functional Rf4 variants and non-functional rf4 variants [15] . Nonetheless, whether the Rf4 locus also underwent copy number variation (CNV) remains unclear. CNV is a significant source of genetic variation, shapes gene expression profiles, and contributes to various adaptive traits in plants [27] , [28] . CNV of genes usually affects gene expression via a gene dosage effect (i.e. more copies of the gene produce more transcripts, which then produce more protein), thus affecting phenotype [29] , [30] . For example, CNV in the GL7 locus in rice affects grain size [31] . CNV of TdDof controls hollow- and solid-stemmed structure in different wheat ( Triticum spp.) species [32] . CNV at the WUS1 locus and the Fas1 locus controls the fate of inflorescence stem cells in maize ( Zea mays ) [33] , [34] . In sugar beet ( Beta vulgaris ), gene dosage of the semidominant locus Rf1 (heterozygotes and homozygotes) affect fertility restoration [35] . Although different CNVs have dosage effects on different agronomic traits in crops [36] , [37] , to date, whether CNV-mediated gene dosage of Rf genes affects fertility restoration remains unclear. In this work, we investigate the origin and evolution of Rf4 in numerous wild rice accessions, landraces, and cultivars. We identify diverse structural variations (SV) and CNV at the Rf4 locus. We find that the CNV of functional Rf4 contributes to fertility restoration of CMS-WA in a dosage-dependent manner. We also reveal the evolutionary history of the Rf4 locus and the co-evolution of Rf4 haplotypes and the CMS gene WA352c . In addition, we develop a set of molecular markers for screening desirable Rf4 haplotypes for breeding. Our findings refine our understanding of the evolutionary plasticity of the Rf genes and the formation of the CMS/ Rf systems, which may accelerate the breeding of elite rice varieties as strong restorer lines for hybrid rice production. Identification of variants and haplotypes of the Rf4 locus in rice cultivars Our and others previous studies identified five variants at the Rf4 locus, namely, Rf4 M and Rf4 I (in indica fertile restorer lines), rf4aus (in circum- aus rice, see below), rf4i (in indica CMS-WA/maintainer lines), and rf4j (in japonica rice) [15] , [17] , [18] . To further reveal the origin and evolution of the Rf4 locus, we re-analyzed the genome sequences of the Rf4 locus using publicly available rice genome information for ZS97B (Zhenshan97B, a maintainer line with rf4i ) ( http://rice.hzau.edu.cn/rice_rs3/ ) [23] , Nip (Nipponbare, a japonica line with rf4j ) ( https://rapdb.dna.affrc.go.jp/ ) [38] , [39] , and MH63 [23] and SH498 ( https://www.mbkbase.org/rice ) [40] (Shuhui498, fertility restorer line carrying functional Rf4 ). We focused on part of a PPR cluster that includes the Rf4 locus based on the reference genome of the restorer line MH63 (Fig. 1a ). Fig. 1: Genomic structure variations and haplotypes at the Rf4 locus. a Homologous gene relationship (microsynteny block) at the Rf4 locus in O. sativa ssp. indica and O. sativa ssp. japonica . b Different haplotypes of the Rf4 complex locus region involving in the Rf4a -copy (Copy-a) and Rf4b -copy (Copy-b) identified in Asian cultivated rice. Gray background shows other PPR genes, white background shows non-functional rf4 variants, black background shows functional Rf4 variants. j : japonica , aus : circum- aus, i : indica , I: IR24, M: MH63, Nip: Nipponbare (a japonica variety). IR24 and MH63 are indica restorer lines. Full size image At the Rf4 locus region, we first examined two lines that lack the ability to restore fertility and identified three PPR genes ( PPR7 [ Os10g0495400 ], rf4j [ Os10g0495200 ], and PPR10 [ Os10g0495100 ]) in Nip (Fig. 1a ) and three PPR genes ( PPR7 , rf4i , PPR10 ) in ZS97B (Fig. 1a ). The rf4i variant was pseudogenized and non-functional due to the presence of a premature termination codon (Fig. 1a ). We next examined two lines that have the ability to restore fertility. The Rf4 locus regions of MH63 and SH498 possess seven PPR genes, in addition to previously known functional Rf4 variant (here defined as Rf4a , of functional Rf4 in Copy-a site of Rf4 locus), PPR 7 , PPR8 , and three copies of PPR10 genes, which included another functional Rf4 variant Rf4b identified in the Copy-b site of Rf4 locus (Fig. 1a ). The interval between Rf4a and Rf4b is 74.8 kb, and the Rf4a and Rf4b coding sequences show 100% amino acid identity. The regions 7.5 kb upstream of the start codon and 1.5 kb downstream of the stop codon of Rf4a and Rf4b showed 98.4% and 99.7% similarity, respectively (Supplementary Data 1 ). These findings reveal that different rice varieties show SV and CNV at the Rf4 locus. Then, we further investigated SV and CNV at the Rf4 locus region in 311 rice cultivars by PCR amplification and sequencing. 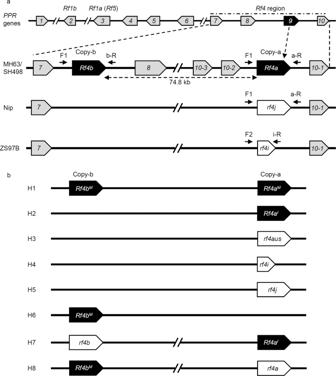Fig. 1: Genomic structure variations and haplotypes at theRf4locus. aHomologous gene relationship (microsynteny block) at theRf4locus inO. sativassp.indicaandO. sativassp.japonica.bDifferent haplotypes of theRf4complex locus region involving in theRf4a-copy (Copy-a) andRf4b-copy (Copy-b) identified in Asian cultivated rice. Gray background shows otherPPRgenes, white background shows non-functionalrf4variants, black background shows functionalRf4variants.j:japonica,aus: circum-aus, i:indica, I: IR24, M: MH63, Nip: Nipponbare (ajaponicavariety). IR24 and MH63 areindicarestorer lines. To this end, we designed site-specific PCR primers based on single-nucleotide polymorphisms (SNPs, Supplementary Table 1 ). The Rf4a and Rf4b genes were amplified using a common primer F1 combined with the site-specific reverse primers a-R and b-R, respectively; the rf4i fragment was amplified using a primer pair F2 and i-R (Fig. 1a ). In total, there were seven variants and eight haplotypes (H1–H8) based on the combination of the Copy-a and Copy-b variants at the Rf4 locus in the modern rice cultivars (Fig. 1b and Supplementary Data 2 ). Sequence analyses demonstrated that the restorer lines contain five haplotypes with one- or two-copy Rf4 variants, including Rf4a I (H2), Rf4b M (H6), Rf4a M -Rf4b M (H1), Rf4a I -rf4b (H7), and rf4a - Rf4b M (H8), while all current CMS-WA lines (and their maintainer lines) carry the rf4i (H4) variant; the rf4j (H5) variant is present mainly in japonica cultivars. Among these variants, rf4aus was previously named as H3 [18] (Fig. 1b ). Diversity and distribution of Rf4 and rf4 variants and haplotypes in the Oryza genus To trace the evolutionary history of Rf4 in the Oryza genus, we further investigated the CNV and sequence polymorphisms of Rf4 and rf4 variants among wild rice and landrace rice accessions. In addition to the seven Rf4 and rf4 variants identified in the cultivars, 61 variants were identified in the Copy-a and/or Copy-b sites of the Rf4 locus (from GG to AA-genome species) (Supplementary Data 2 – 5 ), pointing to the prevalence of SV and CNV in the Rf4 locus. We then performed a BLAST search for putative orthologs and homologs of Rf4 and rf4 in Poaceae genomes in the GenBank database ( https://www.ncbi.nlm.nih.gov/ ). The putative homologs in Aegilops tauschii , Setaria italica , Setaria viridis , Sorghum bicolor , Triticum aestivum , Triticum dicoccoides , and Zea mays were similar to the rice Rf4 and rf4 variants (Supplementary Fig. 1 ). The homologous gene LOC117839145 of S . viridis shared the highest nucleotide sequence similarity of 72.2% with the Rf4 M variants in the rice cultivars (Supplementary Data 6 ). We next used the nucleotide sequences to construct a phylogenetic tree of Rf4 and rf4 in the Oryza genus using LOC117839145 ( S. viridis ) as the outgroup. The variants of different species were divided into six homologous lineages (Supplementary Fig. 2 ). Among these, the rf4i , rf4a , and rf4b clades were closely related to each other, and Rf4 M and Rf4 I were in the same clade, whereas the lineages containing rf4aus and rf4j were closely related (Supplementary Fig. 2 ). During the evolution of wild rice, a considerable number of rf4a , rf4b , and Rf4 variants were developed, but only two variants each of rf4j and rf4i were generated (Supplementary Fig. 2 ). Among Rf4 variants in the different rice cultivars, rf4a , rf4b , rf4aus , rf4i , and Rf4 mainly occur in the indica group, rf4j mainly occurs in the japonica group, and rf4i was only found in bred maintainer lines and CMS-WA lines (Supplementary Data 2 ). In the wild rice O. meyeriana (GG-genome), only a putative one-copy Rf4 variant appeared at the Copy-a site, but not the Copy - b site, thus, this Copy-a variant sequence likely represents the primitive sequence of ancestral Rf4 , which we named Anc-Rf4 (Fig. 2 and Supplementary Data 3 ). Along with sequence variation and genetic recombination, various haplotypes (H13-H68) consisting of Rf4-like and/or rf4-like variants were generated in the genomes of EE ( O. australiensis ), CCDD ( O. alta , O. grandiglumis , and O. latifolia ), CC ( O. eichingeri , O. officinalis , and O. rhizomatis ), BBCC ( O. minuta ), BB ( O. punctata ), and AA genomes ( O. meridionalis , O. glumaepatula , O. rufipogon , and O. nivara ) of these wild species (Fig. 2 and Supplementary Data 3 ); including one-copy haplotypes Rf4a / rf4a-likes (a group of Rf4a-like or rf4a-like variants with SNPs) at the Copy-a site, and Rf4b / rf4b-likes (a group of Rf4b-like or rf4b-like variants with SNPs) at the Copy-b site (H13-H27) (Fig. 2 and Supplementary Data 3 ). Further, various two-copy haplotypes containing Rf4- like and/or rf4- like variants were formed, including Rf4a M -rf4b-likes , rf4a-likes-Rf4b M , rf4a-likes-Rf4b-likes , Rf4a-likes-Rf4b-likes , and rf4a-likes-rf4b-likes (H28-H68) (Fig. 2 and Supplementary Data 3 ). However, no Rf4 and rf4 variants were detected in the tested O. longistaminata , O. barthii , and O. glaberrima accessions at the Copy-a or Copy-b sites (Fig. 2 and Supplementary Data 2 and 3 ). The variants such as rf4i , Rf4a I , and rf4b were first identified in O. australiensis (EE-genome), while Rf4 M and rf4j were first identified in O. officinalis (CC-genome), and rf4aus and rf4a appeared only in indica in O. sativa (Fig. 2 and Supplementary Data 2 – 4 ). Fig. 2: Evolutionary trajectory of Rf4 haplotypes in Oryza species. Current Rf4 haplotypes may have originated from an ancestral type of Rf4 ( Anc-Rf4 , H69), which first emerged at Copy-a in the oldest wild rice O. meyeriana (GG-genome). Sequence variation, gene duplication, and recombination events resulted in new one-copy (H12-H27) or two-copy (H28-H68) haplotypes of R / rf4a-likes (a group of Rf4a-like or rf4a-like variants with SNPs) and/or R / rf4b -likes (a group of Rf4b-like or rf4b-like variants with SNPs) in wild rice. During evolution, along with natural and human selections, the nascent one-copy and two-copy Rf4 and/or rf4 haplotypes gradually migrated into the lineages of O. rufipogon , O. nivara , and O. sativa . Rf4 haplotypes were not detected in tested accessions of O. longistaminata , O. barthii , and O. glaberrima . Among the eight Rf4 haplotypes (H1–H8) in modern cultivars, three two-copy haplotypes (indicated by asterisks “*”, the percentages on the left showed frequency of specific haplotype in the tested accessions) are predominant in restorer lines. H1 ( Rf4a M -Rf4b M ) and H7 ( Rf4a I -rf4b ) haplotypes first appeared in O. nivara and O. australiensis (EE-genome), respectively, while H8 ( rf4a-Rf4b M ) is present only in landraces and modern cultivars of O. sativa . The one-copy variant Rf4a I in H2 of modern cultivars was only found in H7, suggesting that H2 may be derived from loss of rf4b in H7 from O. rufipogon . Other one-copy haplotypes such as H3 ( rf4aus ), H4 ( rf4i ), H5 ( rf4j ) and H6 ( Rf4b M ) first emerged in O. sativa , O. australiensis , O. officinalis (CC-genome), and O. glumaepatula (AA-genome), respectively. The number in the brackets next to each species represents frequency of the haplotypes detected in the species. MYA: million years ago (divergence time). Full size image The rf4 haplotypes are non-functional in restoration of fertility in CMS-WA To confirm the biological functions of the rf4 haplotypes in the rice cultivars, we analyzed amino acid sequence variation among six proteins: rf4a, rf4b, rf4j, rf4aus, Rf4 M , and rf4i. Whereas rf4i is a truncated product containing only eight PPR motifs, the other five proteins contain 18 PPR motifs and share high sequence similarity (93.5–95.3%) (Supplementary Data 7 ). The rf4j, rf4b, rf4aus, and Rf4 M proteins contain 782 amino acids, while rf4a has 798 amino acids (Supplementary Fig. 3 ). In contrast to rf4j vs . Rf4 M , which harbor 37 amino acids differences [15] , [18] , we detected 68 amino acid differences between rf4a and Rf4 M , including two amino acid insertions at the N-terminal regions and 14 amino acid insertions at the C-terminal regions. In addition, rf4b has 38 amino acid differences, and rf4aus harbors 51 amino acid differences to Rf4 M (Supplementary Fig. 3 ). Compared to Rf4 M , all rf4 proteins contain the common 14 amino acid substitutions at the PPR13, PPR14, and PPR15 motifs (Fig. 3a and Supplementary Fig. 3 ), suggesting that amino acid substitutions at these PPRs motifs are important for the fertility restoration of CMS-WA. Fig. 3: Functional characterization of Rf4 haplotypes in cultivated rice. a Amino acid differences used to identify the functional Rf4 and non-functional rf4 variants in three PPR motifs (PPR13, PPR14, and PPR15). b Male fertility of transgenic (T 0 ) lines of Jin23A (a CMS-WA line) carrying different transgenes ( t ) in the hemizygous state. For each complementary construct, at least 10 independent transgenic lines with similar phenotype were obtained. The pollen phenotype of three independent lines was shown in Fig. 3b and Supplementary Fig. 4 . Viable pollen stain black; inviable pollen stain light brown. Scale bar: 50 μm. Full size image To verify our hypothesis that these rf4 variants may be non-functional for fertility restoration, binary vectors containing rf4a , rf4b , rf4j , rf4aus and Rf4 M , all driven by the native promoter from Rf4 , were constructed and introduced into the CMS-WA line Jin23A ( WA352c /H4H4) via transformation. The male fertility of transgenic T 0 plants with the transgene containing Rf4 M was partially restored (Fig. 3b and Supplementary Fig. 4 ). Nevertheless, T 0 transgenic plants carrying rf4a , rf4b , rf4j , or rf4aus remained completely sterile (Fig. 3b and Supplementary Fig. 4 ). These results confirm the notion that all the rf4 haplotypes are non-functional for fertility restoration of CMS-WA. CNV of Rf4 has a dosage effect on fertility restoration of CMS-WA We demonstrated that the Rf4 locus has undergone CNV in different rice cultivars, and assumed that CNV at the Rf4 locus may be associated with the effect on fertility restoration of CMS-WA. To verify the CNV-mediated gene dosage effect of Rf4 , we produced various lines with different copy numbers of Rf4 by crossing Jin23A ( WA352c /H4H4) with two near-isogenic lines of Rf4 : ZSRf4I ( WA352c /H7H7) and ZSRf4M ( WA352c /H1H1), knocking out Rf4 in ZSRf4M lines, and transforming Jin23A with functional Rf4 , respectively (Figs. 4 , 5 and Supplementary Figs. 5 , 6 ). Firstly, the pollen viability (assessed by staining with I 2 –KI) of the F 1 plants derived from Jin23A×ZSRf4I ( WA352c /H4H7) and Jin23A×ZSRf4M ( WA352c /H4H1) were ~71% and ~88%, respectively, while the seed setting rates of these F 1 plants were ~34% and ~52%, respectively (Fig. 4a and Supplementary Figs. 5a , 7a , b ), showing the male fertility of the two-copy Rf4 -carrying plants was higher than those of the one-copy Rf4 -carrying plants (Fig. 4 and Supplementary Figs. 5 , 7 ). Moreover, the fertile anthers were pollen-filled and yellowish, while the sterile anthers appeared thin and whitish (Figs. 4 , 5 and Supplementary Figs. 5 , 6 ). Fig. 4: Validation of the dosage effect of Rf4 using Rf4 near-isogenic lines. a , b Pollen viability based on staining (upper panels), anther phenotype (middle panels), and seed setting rate (lower panels) of Jin23A×ZSRf4I ( WA352c /H4H7), Jin23A×ZSRf4M ( WA352c /H4H1) and rf4a m -rf4b m -mF 1 / rf4a m -rf4b m mutant lines (by CRISPR/Cas9 editing) in the ZSRf4M background. Red “×” indicates the non-functional rf4a / b m after knockout of Rf4a / b M . Scale bars: 50 μm in the upper panels, 1 cm in the middle panels, and 5 cm in the lower panels. c – e Transcript levels of Rf4 ( c ) and WA352c ( d , e ) in different lines. UFC1 ( UFM1-Conjugating Enzyme 1 ) and atp6 (a mitochondrial gene) served as internal references for Rf4 and WA352c expression, respectively. Data are shown as mean ± SD, n = 3 biological replicates. Significant differences between two samples were determined by two-tailed Student’s t -test (** P <  0.01, *** P <  0.001, **** P <  0.0001). f Sequencing of the Rf4a / b M -knockout plants derived from CRISPR/Cas9 editing. The underlined bases show protospacer adjacent motifs (PAMs). The positions highlighted in red indicate the targeted mutations. Source data are provided as a Source data file. Full size image Fig. 5: Confirmation of the dosage effect of Rf4 in complemention lines. a Pollen staining (upper panels) to reveal viable pollen (dark), anther phenotype (middle panels) and seed setting rate (lower panels) of Jin23A/ Rf4 t - ( WA352c /H4 Rf4 t -), Jin23A/ Rf4 t Rf4 t ( WA352c /H4H4 Rf4 t Rf4 t ), and Jin23A/ Rf4 t Rf4 t ×ZSRf4I ( WA352c /H4H7 Rf4 t - ). Scale bars: 50 μm in the upper panels, 1 cm in the middle panels, and 5 cm in the lower panels. b , c Transcript levels of Rf4 ( b ) and WA352c ( c ) in different lines. “ Rf4 t ” indicates the Rf4 transgene, “ Rf4 t - ” indicates transgenic hemizygotes. Data are shown as mean ± SD, n = 3 biological replicates. Significant differences between two samples were determined by two-tailed Student’s t -test (** P <  0.01, *** P <  0.001, and NS represents No Significance). Source data are provided as a Source data file. Full size image Furthermore, we knocked out both Rf4a M and Rf4b M in ZSRf4M line by CRISPR/Cas9 editing and obtained several rf4a m and rf4b m mutants, which showed full abortion of pollen and spikelet (Fig. 4b , Supplementary Fig. 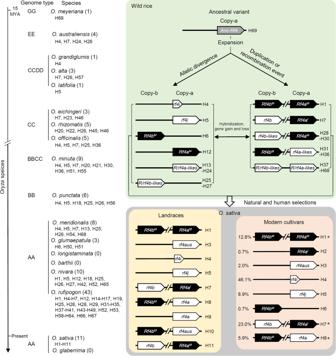Fig. 2: Evolutionary trajectory ofRf4haplotypes inOryzaspecies. CurrentRf4haplotypes may have originated from an ancestral type ofRf4(Anc-Rf4, H69), which first emerged at Copy-a in the oldest wild riceO. meyeriana(GG-genome). Sequence variation, gene duplication, and recombination events resulted in new one-copy (H12-H27) or two-copy (H28-H68) haplotypes ofR/rf4a-likes(a group ofRf4a-likeorrf4a-likevariants with SNPs) and/orR/rf4b-likes (a group ofRf4b-likeorrf4b-likevariants with SNPs) in wild rice. During evolution, along with natural and human selections, the nascent one-copy and two-copyRf4and/orrf4haplotypes gradually migrated into the lineages ofO. rufipogon,O. nivara, andO. sativa.Rf4haplotypes were not detected in tested accessions ofO. longistaminata,O. barthii, andO. glaberrima. Among the eightRf4haplotypes (H1–H8) in modern cultivars, three two-copy haplotypes (indicated by asterisks “*”, the percentages on the left showed frequency of specific haplotype in the tested accessions) are predominant in restorer lines. H1 (Rf4aM-Rf4bM) and H7 (Rf4aI-rf4b) haplotypes first appeared inO. nivaraandO. australiensis(EE-genome), respectively, while H8 (rf4a-Rf4bM) is present only in landraces and modern cultivars ofO. sativa. The one-copy variantRf4aIin H2 of modern cultivars was only found in H7, suggesting that H2 may be derived from loss ofrf4bin H7 fromO. rufipogon. Other one-copy haplotypes such as H3 (rf4aus), H4 (rf4i), H5 (rf4j) and H6 (Rf4bM) first emerged inO. sativa,O. australiensis,O. officinalis(CC-genome), andO. glumaepatula(AA-genome), respectively. The number in the brackets next to each species represents frequency of the haplotypes detected in the species. MYA: million years ago (divergence time). 5b , and Supplementary Table 2 ). Then, we selected three rf4a m and rf4b m loss-of-function mutant lines (carrying different editing patterns) and crossed them with wild type ZSRf4M to test the dosage effect of Rf4 in the resultant mutant F 1 (mF 1 ) (Fig. 4b and Supplementary Fig. 5b ). As expected, the pollen and spikelets of mF 1 plants carrying two copies of Rf4 ( WA352c /H1h1) also showed lower pollen viability (~85%) and seed setting rate (~48%), compared to those of wild type ZSRf4M (~92% and ~72%, respectively), which carries four copies of Rf4 (Fig. 4b and Supplementary Figs. 5b , 7c , d ). To clarify the connection between the Rf4 CNV-mediated gene dosage effect and the WA352c repression in fertility restoration, we performed qRT-PCR analysis of Rf4 and WA352c expression in anthers of different plants at the microspore mother cell stage. The expression level of Rf4 was twice as high in Jin23A×ZSRf4M ( WA352c / H4H1) vs . Jin23A×ZSRf4I ( WA352c /H4H7) (Fig. 4c and Supplementary Fig. 5c ), whereas the expression pattern of WA352c was opposite to that of Rf4 (Fig. 4d and Supplementary Fig. 5d ). The level of WA352c transcripts was higher in the rf4a m -rf4b m -mF 1 and rf4a m -rf4b m lines compared to ZSRf4M (Fig. 4e and Supplementary Fig. 5e ). In addition, we generated Rf4 t - transgenic lines using CMS line Jin23A as recipient and selected a homozygous Jin23A/ Rf4 t Rf4 t ( WA352c /H4H4 Rf4 t Rf4 t ) plant from the T 1 population to cross with ZSRf4I generating F 1 plants Jin23A/ Rf4 t Rf4 t ×ZSRf4I ( WA352c /H4H7 Rf4 t - ). We then acquired a series of materials harboring different copy numbers of the Rf4 t transgene in the F 2 population. As expected, lines with two-copy Rf4 , including Jin23A/ Rf4 t Rf4 t ( WA352c /H4H4 Rf4 t Rf4 t ) and Jin23A/ Rf4 t Rf4 t ×ZSRf4I ( WA352c /H4H7 Rf4 t - ), exhibited higher pollen viability (~87%, ~90%) and spikelet fertility (~52%, ~53%) than J23A/ Rf4 t - lines harboring a single copy of Rf4 ( WA352c /H4H4 Rf4 t - ), which showed ~73% pollen fertility and ~36% spikelet fertility (Fig. 5a and Supplementary Figs. 6a , 7e , f ). The level of Rf4 transcripts in Jin23A/ Rf4 t Rf4 t ( WA352c /H4H4 Rf4 t Rf4 t ) and Jin23A/ Rf4 t Rf4 t ×ZSRf4I ( WA352c /H4H7 Rf4 t - ) was about twice as high as that in Jin23A/ Rf4 t - ( WA352c /H4H4 Rf4 t - ) in qRT-PCR assays (Fig. 5b and Supplementary Fig. 6 ). Consistent with this, the pattern of WA352c transcript levels was opposite to that of Rf4 (Fig. 5c and Supplementary Fig. 6c ). Together, these results supported the hypothesis that the dosage effect caused by different copy number of functional Rf4 plays an important role in fertility restoration of CMS-WA. The haplotypes with two-copy functional Rf4 are widely used in three-line hybrid rice breeding The ability to restore fertility of CMS lines restricts hybrid rice production; therefore, genetic resources with two-copy Rf4 might be beneficial for breeding stronger restorer lines for CMS-WA in hybrid rice production. To investigate the relationship between haplotypes of the Rf4 locus and the application of major restorer lines in China, we obtained data about the planting areas of hybrid rice varieties and crossing combinations of restorer lines for CMS-WA from the China Rice Data Center ( https://www.ricedata.cn/ ). 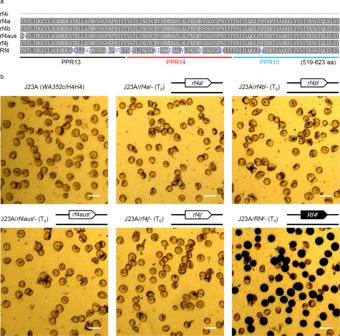Fig. 3: Functional characterization ofRf4haplotypes in cultivated rice. aAmino acid differences used to identify the functional Rf4 and non-functional rf4 variants in three PPR motifs (PPR13, PPR14, and PPR15).bMale fertility of transgenic (T0) lines of Jin23A (a CMS-WA line) carrying different transgenes (t) in the hemizygous state. For each complementary construct, at least 10 independent transgenic lines with similar phenotype were obtained. The pollen phenotype of three independent lines was shown in Fig. 3b and Supplementary Fig.4. Viable pollen stain black; inviable pollen stain light brown. Scale bar: 50 μm. With regards to planting area of three-line hybrid rice cultivars, we selected the top sixteen related restorer lines for analysis: six lines (MH63, Ce64-7, CDR22, FuHui838, MH86, and ChengHui727) carried H1 ( Rf4a M -Rf4b M ), eight lines (MiYang46, Gui99, IR24, R402, Shuhui527, Huazhan, Guanghui998, and Minhui3301) harbored H7 ( Rf4a I -rf4b ), XianHui207 contained H8 ( rf4a-Rf4b M ), and MianHui725 possessed H6 ( Rf4b M ) (Supplementary Table 3 ). As expected, hybrid rice varieties using six restorer lines carrying two-copy Rf4 (H1) had a larger total planting area (135,998,667 hectares) than the hybrid rice varieties using ten restorer lines having the one-copy Rf4 (78,015,332 hectares) (Fig. 6 ). Notably, the two most widely planted hybrid rice varieties were bred from two elite restorer lines, MH63 and Ce64-7, both carrying the two-copy Rf4 (Supplementary Table 3 ). Fig. 6: Usage of Rf4 haplotypes in major restorer lines for hybrid rice production in China. Total planting areas and relative percentage of hybrid rice varieties in China using 6 restorer lines carrying the two-copy Rf4 (H1) and 10 restorer lines with one-copy Rf4 (H6, H7, H8). The data information is given in Supplementary Table 3 . Full size image The rf4i variant is dominantly used for the breeding of CMS-WA lines The rice mitochondrial CMS-WA gene WA352c was generated in O. rufipogon via multiple rounds of recombination/protogene formation/functionalization, and WA352c has been widely utilized in hybrid rice breeding [1] . However, how WA352c co-evolved with Rf4 remains to be uncovered. To explore the evolutionary relationship of WA352c with Rf4 , we analyzed their sequence structures in different O. rufipogon species and rice cultivars. The functional WA352c gene only coexisted with three haplotypes (H7, H14, and H28) of the Rf4 locus in O. rufipogon populations (Table 1 ). This finding suggests that the first CMS-WA germplasm with abortive pollen discovered from an O. rufipogon population, called Wild Abortive, carrying a rf4a-like variant in addition to WA352c (Fig. 7 , Table 1 ). Table 1 Association of WA352c and Rf4 haplotypes in different populations of O. rufipogon and O. sativa Full size table Fig. 7: A speculative model for formation of the CMS-WA/ Rf system. An Oryza rufipogon population (Wild Abortive) with the mitochondrial sterility gene WA352c and non-functional rf4a-like showing pollen abortion was found and used as the female parent for breeding CMS-WA lines by backcrossing with indica maintainer lines containing rf4i . A hybrid rice variety was bred by crossing the CMS-WA line with a restorer line (carrying one-copy or two-copy Rf4 ). Full size image During the process of CMS-WA line breeding, the rf4a-like variant was replaced by rf4i through backcrossing with indica maintainer lines that harbor the rf4i variant, resulting in the current CMS-WA lines (Fig. 7 , Table 1 ). CMS-WA ( WA352c / rf4irf4i ), maintainer ( rf4i ), and restorer lines ( Rf4 ) made up the CMS-WA/ Rf system for three-line hybrid rice production (Fig. 7 ). Based on the above results and the previous finding that WA352c originates in O. rufipogon [1] , it appears that Rf4 and rf4 (except for rf4a and rf4aus ) originated earlier than WA352c (Fig. 7 , Table 1 , and Supplementary Data 3 ) and that the replacement of rf4i derived from indica type maintainer lines occurred during the creation of modern CMS-WA lines. PCR-based molecular markers for genotyping the Rf4 locus to assist hybrid rice breeding To facilitate the identification of Rf4 ( rf4 ) haplotypes in hybrid rice breeding, we selected and optimized a set of eight Rf4 variant-specific PCR-based markers based on the SNPs at the Rf4 locus (Supplementary Table 1 ). To confirm the utility of this set of markers, these primers were used to investigate the genotypes of 304 Asian cultivated rice germplasms. PCR products of these lines were first divided into three types, Copy-a, Copy-b, and Copy-a/-b, using two PCR markers (Copy-a-332 bp-F/R and Copy-b-282 bp-F/R), which generated 332-bp- and 282-bp PCR products from Copy-a and Copy-b, respectively (Fig. 8 and Supplementary Table 1 ). Then the variants and haplotypes of Rf4 and rf4 were determined using six specific primer sets. The fragments amplified from one-copy Rf4 from the Copy-a or Copy-b in rice varieties with the Rf4a I haplotype (such as Jalmagna and GH102) or Rf4b M haplotype (such as MH725 and R60) were 262 bp long (Fig. 8a ). No products of functional Rf4 were amplified from japonica , indica , and aus varieties carrying haplotypes of rf4j, rf4i , and rf4aus , but a 372-bp, 358-bp, and 351-bp products of rf4 were obtained from the Copy-a of these varieties, respectively (Fig. 8b ). Fig. 8: Identifying different Rf4 haplotypes in cultivated rice. Eight pairs of variant-specific primers were used for PCR to determine the Rf4 and rf4 haplotypes of different rice lines. a One-copy Rf4 , b one-copy rf4 , c two-copy Rf4 . White dashed lines separate four different patterns of one-copy Rf4 . GH993 (Guanghui993), XH207 (Xianhui207), ZSRf4I (Zhenshan Rf4I), IR8, Jalmagna, GH102 (Guanghui 102), MH725 (Mianhui725), R60, J23 (Jin23), ZS97 (Zhenshan97), IR64, 9311, MH63 (Minghui63), SH498 (Shuhui498), FH838 (Fuhui838), and IR30 are indica cultivars. Nip, T65, ZH11, and 9522 are japonica cultivars. CISOKAN, BaXiang, AR (Albania Rice), and ZCD13 (Zacaodao13) are circum- aus cultivars. Actin1 was used as the PCR control. The PCR experiments for each sample were independently repeated at least three times with similar results. Source data are provided as a Source data file. Full size image Varieties with the rf4a - Rf4b M haplotype (such as GH993 and XH207) or the Rf4a I - rf4b haplotype (such as ZSRf4I and IR8) all carried one-copy Rf4 (Fig. 8a ). They shared four common PCR products: Copy-a (332 bp), Copy-b (282 bp), Rf4 (262 bp), and rf4a / b (197 bp). Varieties with the rf4a - Rf4b M haplotype also generated another product: rf4a (446 bp). Varieties carrying two-copy Rf4 with the Rf4a M - Rf4b M haplotype (such as MH63, SH498, FH838, and IR30) generated three PCR products: Rf4 (262 bp), Copy-a (332 bp), and Copy-b (282 bp) (Fig. 8c ). Taken together, these results demonstrated that these primer sets are useful PCR markers for the rapid genotyping to accelerate the screening of strong restorer lines with the two-copy Rf4 . The CMS/ Rf system has been widely used in hybrid seed production [41] , [42] . Functional CMS genes originated and evolved via a multiple recombination, protogene formation, and complex diversification [1] , [43] . However, our understanding of Rf gene evolution and its co-evolution with CMS genes is very limited. Here, we demonstrated the evolutionary plasticity of Rf4 in terms of sequence structure, copy number, and biological function during the evolution of the Oryza genus. Structural variation (duplications, deletions, insertions, and chromosomal rearrangements) is an important driver of phenotypic variability in crop traits during the processes of evolution and domestication [28] , [44] , [45] . Based on public genome information for rice and sequencing of PCR products, we reconstructed a diagram of the genetic structure of the Rf4 complex locus in three rice varieties (Fig. 1a ) and its genetic structure in different rice cultivars. We discovered that the Rf4 locus shows CNV associated with the restoration effect of this locus. In total, eight haplotypes were identified in modern rice cultivars, including the two-copy haplotypes such as H1 ( Rf4a M -Rf4b M ), H7 ( Rf4a I -rf4b ), and H8 ( rf4a-Rf4b M ), as well as the one-copy haplotypes such as H2 ( Rf4a I ), H3 ( rf4aus ), H4 ( rf4i ), H5 ( rf4j ), and H6 ( Rf4b M ) (Fig. 1b ). The functional Rf4 variants enabled the degradation of WA352c transcripts through post-transcriptional mechanism and restore the male fertility of CMS-WA, whereas rf4a , rf4b , rf4aus , and rf4j are non-functional variants like rf4i (Fig. 3b and Supplementary Fig. 4 ). Furthermore, our findings indicated that the functionalization of Rf4 protein is affected by 14 amino acids in three motifs from PPR13 to PPR15 (Fig. 3 ). How these amino acids determine the fertility restoration activity of the protein requires further study. Rf genes identified in plants mainly encode a subclass of PPR proteins that are subjected to rapid evolution [20] , [46] . The rice Rf loci encoding PPR proteins show considerable structural and sequence variation within and among Oryza species [22] , [47] . In this study, we revealed that the ancestral Rf4 -like sequence first appears at the “Copy-a” site of the Rf4 locus in O. meyeriana (GG-genome), which is regarded as the oldest wild rice species. Subsequently, the Rf4 locus likely experienced more expansions in the genome of multiple wild rice species, leading to the sequence variation and duplication of Rf4 or rf4 in the Copy-a and/or Copy-b sites (Fig. 2 and Supplementary Data 3 ). One-copy haplotypes of Rf4 might have appeared early in the evolution of the Oryza genus, and different haplotypes of Rf4 might have multiple origins and co-exist in the wild rice gene pool. Based on the 68 variants identified from the Copy-a and/or Copy-b sites, and 69 haplotypes at the Rf4 locus, we reasoned that the Rf4 locus shows high plasticity in Oryza (Fig. 2 and Supplementary Fig. 2 ). During evolution, along with natural and human selections, the nascent one-copy and two-copy Rf4 haplotypes gradually migrated into the lineages of O. rufipogon , O. nivara , and O. sativa , and finally became enriched in modern Asian cultivars. However, the Rf4 gene flow might have failed to pass through certain bottleneck events to enter the lineages of O. longistaminata , O. barthii , and O. glaberrima , so the Rf4 haplotypes were not detected in the tested accessions. Alternatively, considerable structural and sequence variations might occur in the lineages of O. longistaminata , O. barthii , and O. glaberrima , leading to gene loss in the Rf4 locus (Fig. 2 ). Notably, there are only eight Rf4 haplotypes (H1–H8) enriched in modern rice cultivars, and the two-copy Rf4 haplotypes (H1) are predominant in three-line hybrid rice varieties (Fig. 6 ). Among the eight Rf4 haplotypes, five are widely distributed in the wild rice accessions, suggesting that these haplotypes might have preexisted in different wild rice species (Fig. 2 and Supplementary Data 3 ). Since the Rf4a I variant is only detected in the one-copy H2 ( Rf4a I ) in modern cultivars and the two-copy H7 ( Rf4a I -rf4b ) in wild rice species; the H2 might have directly originated from H7 due to loss of rf4b during domestication (Fig. 2 ). Gene dosage effects caused by CNV are always accompanied by changes in gene expression levels and protein accumulation. These processes are involved in human diseases and agricultural traits in both animals and plants [36] , [48] . We found that the Rf4 complex locus had different forms of CNV, which resulted in a gene dosage effect. Varieties or hybrids carrying two/four copies of Rf4 showed higher pollen fertility, full anthers, and higher seed setting rates than those carrying one/two copies of Rf4 (Figs. 4 a, b, 5a and Supplementary Figs. 5a , b , 6a ). By contrast, the level of WA352c transcript decreased with increasing copy of Rf4 (Figs. 4 c–e, 5 b, c and Supplementary Figs. 5c – e , 6b , c ). We also investigated the application of Rf4 haplotypes in three-line hybrid rice production in China. As expected, restorer lines containing two-copy Rf4 (such as MH63, FH838, etc.) had larger planting areas than restorer lines carrying one-copy Rf4 (such as MiYang46, Gui99, etc.) (Fig. 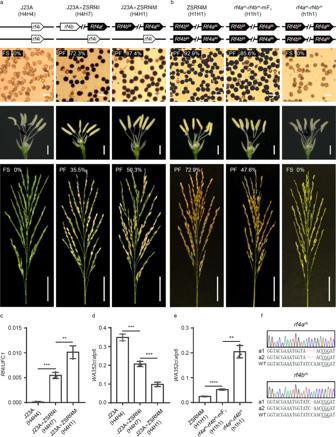Fig. 4: Validation of the dosage effect ofRf4usingRf4near-isogenic lines. a,bPollen viability based on staining (upper panels), anther phenotype (middle panels), and seed setting rate (lower panels) of Jin23A×ZSRf4I (WA352c/H4H7), Jin23A×ZSRf4M (WA352c/H4H1) andrf4am-rf4bm-mF1/rf4am-rf4bmmutant lines (by CRISPR/Cas9 editing) in the ZSRf4M background. Red “×” indicates the non-functionalrf4a/bmafter knockout ofRf4a/bM. Scale bars: 50 μm in the upper panels, 1 cm in the middle panels, and 5 cm in the lower panels.c–eTranscript levels ofRf4(c) andWA352c(d,e) in different lines.UFC1(UFM1-Conjugating Enzyme 1) andatp6(a mitochondrial gene) served as internal references forRf4andWA352cexpression, respectively. Data are shown as mean ± SD,n= 3 biological replicates. Significant differences between two samples were determined by two-tailed Student’st-test (**P<  0.01, ***P<  0.001, ****P<  0.0001).fSequencing of theRf4a/bM-knockout plants derived from CRISPR/Cas9 editing. The underlined bases show protospacer adjacent motifs (PAMs). The positions highlighted in red indicate the targeted mutations. Source data are provided as a Source data file. 6 and Supplementary Table 3 ), suggesting that stronger capacity for fertility restoration is an important trait selected by breeders. Therefore, rice materials carrying the two-copy Rf4 ( Rf4a M -Rf4b M ) were preferentially selected by breeders to generate strong restorer lines for three-line hybrid rice production. Notably, Rf4 is located in a hotspot of a Rf gene cluster on Chromosome 10 in rice, and clusters with other restorer genes including Rf1a / Rf5 for CMS-BT/CMS-HL, Rf1b for CMS-BT [24] , [25] , and Rf19 for CMS-FA [26] . Pyramiding multiple restorer genes in a restorer line can expand the crossbreeding combinations and increase planting area of related hybrid varieties. In general, Rf or Rf-like genes show certain characteristic features, including genomic clustering and unique evolutionary patterns [19] , [20] , [22] . Functional Rf4 variants exist in ancient wild rice species (EE- and CC-genome), landrace, and modern cultivars (Fig. 2 , Supplementary Fig. 2 , and Supplementary Data 2 – 4 ), pointing to its evolutionary conservation. Since WA352c is a newly evolved mitochondrial sterility gene in O. rufipogon [1] , Rf4 (and its variants) may have had other undiscovered intrinsic functions prior to its neofunctionalization as a fertility restorer for WA352c during the adaptive evolution of wild rice. Moreover, we determined that all current CMS-WA lines used for hybrid rice production contain the combination of WA352c and rf4i , which is not present in O. rufipogon (Table 1 and Supplementary Data 3 ). H4 ( rf4i ) is a pseudogene due to the insertion of fragments leading to premature termination [15] , which might firstly occur in O. australiensis and might have become predominant in rice landraces (Fig. 2 and Supplementary Data 3 and 4 ). Based on our findings, we suggest that the rf4a-like variant (H14) and WA352c is the original combination in O. rufipogon , which was later termed Wild-Abortive germplasm (Fig. 7 , Table 1 , and Supplementary Data 3 ). In early 1970s in China, this CMS germplasm was explored for breeding CMS-WA lines by backcrossing with recurrent parental ( indica ) varieties (maintainer lines) carrying the rf4i variant (Fig. 7 ). Molecular marker-assisted selection (MAS) is an effective tool for accelerating the screening of crops with desired genotypes [49] , [50] . In this study, we developed a set of precise PCR-based molecular markers to identify Rf4 and rf4 haplotypes at the Rf4 locus. The functional Rf4 variants in a variety could be identified using the Rf4 marker, and CNV of the Rf4 locus could be characterized using four markers: Copy-a, Copy-a, rf4a , and rf4a / b (Fig. 8a, b ). Thus, we recommend that breeders use five markers ( Rf4 , Copy-a, Copy-b, rf4a , and rf4a/b ) to identify germplasm with two-copy Rf4 to generate elite restorer lines (Fig. 8c ). A one-copy rf4 haplotype is present in Copy-a, the japonica and aus varieties harbor the rf4j and rf4aus variants, respectively, while all CMS-WA lines and maintainer lines examined harbor the rf4i variant (Fig. 8b ). Therefore, the rf4i marker is an accurate marker for MAS of new CMS-WA lines and maintainer lines in landrace and/or cultivated rice backgrounds. Rice germplasms carrying the rf4aus and rf4j haplotypes lack the function for fertility restoration (Fig. 3b ), but they have the potential to be new CMS/maintainer lines for future hybrid rice breeding. Meanwhile, landraces and modern Asian rice varieties that carry Rf4 variants (including the one-copy Rf4 and two-copy Rf4 ones) were screened as restorer lines by human selection (Figs. 2 , 7 ). Although breeders may not be aware of the CNV of Rf4 in the breeding programs, they selected successful restorer lines based on their ability of fertility restoration along with other beneficial agronomic traits. We believe that our findings will benefit the high-efficiency breeding of CMS/maintainer lines and restorer lines to improve hybrid rice yields in the future. Plant materials All plant materials were grown in the rice field in South China Agricultural University, Guangzhou, China. The wild rice accessions were selected from “Ding’s Rice Collection” in South China Agricultural University. Landraces and cultivars of O. sativa were collected from different provinces in China and used to examine the haplotypes of Rf4 and rf4 . The CMS-WA line Jin23A served as the recipient for the Rf4 and rf4 functional complementation assays. Near-isogenic lines ZSRf4I and ZSRf4M were derived from backcrosses of the CMS-WA line ZS97A with the restorer line IR24 and MH63, respectively. Vector construction and plant transformation The coding sequences of Rf4 M , rf4a , rf4b , rf4aus , and rf4j driven by the native promoter of Rf4 M and followed by a Nos terminator were cloned into modified pCAMBIA1300 binary vectors by the Gibson assembly method [51] . The CRISPR/Cas9 knockout plasmid for Rf4 was constructed as previously reported [52] . Briefly, target sequence (ggtacgaaatggtatccaac) selected in the coding region of Rf4 were introduced into sgRNA expression cassette by overlapping PCR, then the cassette was cloned into the CRISPR/Cas9 binary vector by the Gibson assembly method [52] . These generated constructs were introduced into Agrobacterium tumefaciens strain EHA105, and then transformed into Jin23A or ZSRf4M by the Agrobacterium tumefaciens -mediated method. Primers for vector construction are listed in Supplementary Table 1 . Genotyping and phenotypic characterization of fertility in the transgenic lines Pollen grains were stained with 1% I 2 -KI solution and imaged under a light microscope (Axio Observer D1, Carl Zeiss, Oberkochen, Germany) to measure the pollen viability rate, and the main panicle was collected from each individual to examine the seed setting rate and photographed with a camera (Canon, Japan). We obtained at least 10 independent transgenic lines for each complementary construct with similar phenotype and showed the phenotype of three independent lines in Fig. 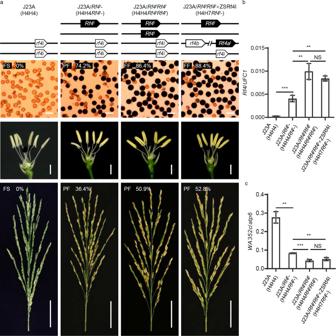Fig. 5: Confirmation of the dosage effect ofRf4in complemention lines. aPollen staining (upper panels) to reveal viable pollen (dark), anther phenotype (middle panels) and seed setting rate (lower panels) of Jin23A/Rf4t- (WA352c/H4Rf4t-), Jin23A/Rf4tRf4t(WA352c/H4H4Rf4tRf4t), and Jin23A/Rf4tRf4t×ZSRf4I (WA352c/H4H7Rf4t-). Scale bars: 50 μm in the upper panels, 1 cm in the middle panels, and 5 cm in the lower panels.b,cTranscript levels ofRf4(b) andWA352c(c) in different lines. “Rf4t” indicates theRf4transgene, “Rf4t-” indicates transgenic hemizygotes. Data are shown as mean ± SD,n= 3 biological replicates. Significant differences between two samples were determined by two-tailed Student’st-test (**P<  0.01, ***P<  0.001, and NS represents No Significance). Source data are provided as a Source data file. 3b and Supplementary Fig. 4 . The flowers and main panicles from ten different plants of each independent line were selected for statistical analysis of pollen viability and seed setting rate, respectively. The T-DNA flanking sequences of Rf4 were identified using mhiTAIL-PCR [53] . T-DNA tags of the transgenic plants were genotyped using specific primer sets. In addition, the genotypes of Rf4 -variants were determined using the Rf4 -linked marker. Four independent Rf4 -knockout plants were genotyped through PCR-based sequencing. Primers used for genotyping complementary or knockout lines are listed in Supplementary Table 1 . PCR-based haplotype analysis Molecular markers (Supplementary Table 1 ) were designed based on sequence differences among the Copy-a, Copy-b, Rf4 , rf4a , rf4a / b , rf4i , rf4aus , and rf4j to identify the haplotypes of Rf4 and rf4 in cultivated rice by PCR. Each 20 μL reaction contained 10 μL 2× Taq PCR StarMix with Loading Dye (Genstar, China), 0.125–0.25 mM primer, and 1 μL DNA (50–100 ng). PCR was performed under the following conditions: 94 °C for 4 min; 29 cycles of 94 °C for 30 s, 59 °C for 30 s, and 72 °C for 20 s; a final extension of 2 min at 72 °C. Long DNA fragments of the Copy-a and Copy-b were amplified with specific primers using STI PCR [54] . The amplified DNA fragments were sequenced and analyzed by BLAST ( http://www.ncbi.nlm.nih.gov/BLAST/ ) and Clustal Omega ( https://www.ebi.ac.uk/Tools/msa/clustalo/ ). Sequencing of WA352c was performed using previously described primers [15] . All the PCR experiments for each sample were performed with at least three replicates. 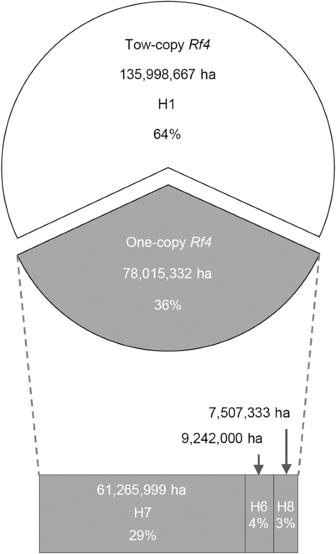Fig. 6: Usage ofRf4haplotypes in major restorer lines for hybrid rice production in China. Total planting areas and relative percentage of hybrid rice varieties in China using 6 restorer lines carrying the two-copyRf4(H1) and 10 restorer lines with one-copyRf4(H6, H7, H8). The data information is given in Supplementary Table3. The PCR products were separated on 1.5–2% agarose gels by conventional electrophoresis. RNA extraction and qRT-PCR analysis Total RNA was extracted from rice anthers at the microspore mother cell stage [55] using TRIzol reagent (Ambion, USA), followed by reverse transcription into cDNA using a HiScript III 1 st Strand cDNA Synthesis Kit (Vazyme, China) with oligo(dT) and random hexamers according to the manufacturer’s instructions. qRT-PCR analysis was performed on the Bio-Rad CFX Real-Time PCR system (Bio-Rad, USA). Expression analysis of Rf4 and WA352c was performed by qRT-PCR with specific primers (Supplementary Table 1 ) with three biological replicates; UFC1 (encoding a homolog of UFM1-Conjugating Enzyme 1, GenBank number: AK059551), which is a constitutive expression gene with medium level suitable as internal reference gene [56] , and atp6 (the mitochondrial gene encoding a subunit of ATP synthase) [15] , were used as internal controls for the expression of Rf4 and WA352c , respectively. Phylogenetic and evolutionary analyses of the Rf4 locus The orthologs of Rf4 in the Poaceae family were identified for phylogenetic analysis of Rf4 using the tblastn program in the GenBank database ( https://www.ncbi.nlm.nih.gov/ ) based on the Rf4 sequence in the cultivars. To trace the divergence and perform phylogenetic analysis of the Rf4 locus, Rf4 and rf4 fragments were amplified and sequenced in all wild rice, landrace, and cultivated rice accessions with specific primers (Supplementary Table 1 ). The nucleotide sequences of Rf4 homologs were aligned with MAFFT v.7.475 [57] and manually adjusted using MEGA X v.10.1.7 [58] . Phylogenetic analysis was conducted using the maximum likelihood method with MEGA X v.10.1.7. Bootstrapping with 1000 replicates was used to generate the best tree and its branches. The phylogenetic trees were then plotted with the online tool Interactive Tree of Life ( https://itol.embl.de/ ). 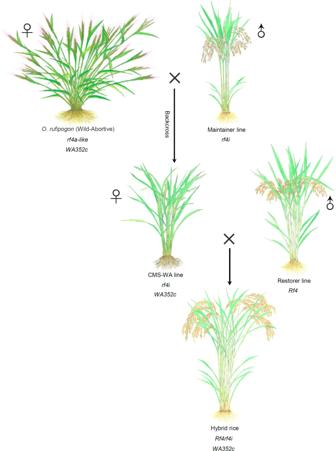Fig. 7: A speculative model for formation of the CMS-WA/Rfsystem. AnOryza rufipogonpopulation (Wild Abortive) with the mitochondrial sterility geneWA352cand non-functionalrf4a-likeshowing pollen abortion was found and used as the female parent for breeding CMS-WA lines by backcrossing withindicamaintainer lines containingrf4i. A hybrid rice variety was bred by crossing the CMS-WA line with a restorer line (carrying one-copy or two-copyRf4). 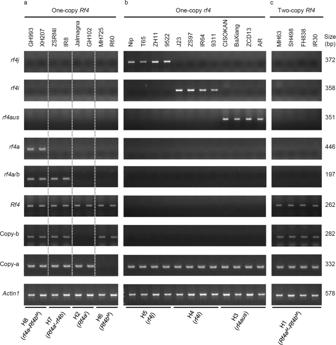Fig. 8: Identifying differentRf4haplotypes in cultivated rice. Eight pairs of variant-specific primers were used for PCR to determine theRf4andrf4haplotypes of different rice lines.aOne-copyRf4,bone-copyrf4,ctwo-copyRf4. White dashed lines separate four different patterns of one-copyRf4. GH993 (Guanghui993), XH207 (Xianhui207), ZSRf4I (Zhenshan Rf4I), IR8, Jalmagna, GH102 (Guanghui 102), MH725 (Mianhui725), R60, J23 (Jin23), ZS97 (Zhenshan97), IR64, 9311, MH63 (Minghui63), SH498 (Shuhui498), FH838 (Fuhui838), and IR30 areindicacultivars. Nip, T65, ZH11, and 9522 arejaponicacultivars. CISOKAN, BaXiang, AR (Albania Rice), and ZCD13 (Zacaodao13) are circum-auscultivars.Actin1was used as the PCR control. The PCR experiments for each sample were independently repeated at least three times with similar results. Source data are provided as a Source data file. Reporting summary Further information on research design is available in the Nature Portfolio Reporting Summary linked to this article.